Correlated loss of ecosystem services in coupled mutualistic networks Networks of species interactions promote biodiversity and provide important ecosystem services. These networks have traditionally been studied in isolation, but species are commonly involved in multiple, diverse types of interaction. Therefore, whether different types of species interaction networks coupled through shared species show idiosyncratic or correlated responses to habitat degradation is unresolved. Here we study the collective response of coupled mutualistic networks of plants and their pollinators and seed dispersers to the degradation of Europe’s last relict of old-growth lowland forest (Białowieża, Poland). We show that logging of old-growth forests has correlated effects on the number of partners and interactions of plants in both mutualisms, and that these effects are mediated by shifts in plant densities on logged sites. These results suggest bottom-up-controlled effects of habitat degradation on plant–animal mutualistic networks, and predict that the conversion of primary old-growth forests to secondary habitats may cause a parallel loss of multiple animal-mediated ecosystem services. All species are directly or indirectly involved in mutualistic and antagonistic interactions that together form complex interaction networks [1] , [2] . These networks of species interactions structure ecological communities [3] and maintain processes that are essentially linked to the functioning of ecosystems [4] . Recent studies provide evidence that the structure of such networks is altered by habitat degradation [5] , and that rare and specialized interactions are the first to disappear after habitat reduction [6] . However, to date, most studies have focussed on only a single type of interaction (for example, pollination) even though species are commonly involved in multiple, diverse types of interaction [2] , [7] . A key question is hence whether habitat degradation has correlated effects on multiple interaction networks each providing different ecosystem services, such as pollination and seed dispersal [4] , [7] . For example, a correlated response to habitat degradation could arise through the sharing of plant resources among different interaction networks [7] , [8] , [9] . Simulations suggest that extinction of plants can cause correlated co-extinctions in different interaction networks when these are coupled through shared plant resources [7] . This implies that plants are critical nodes of coupled interaction networks [7] , [9] , and that plants may mediate a correlated response of such coupled networks to habitat degradation. Here we empirically test this prediction on coupled mutualistic networks of 10 keystone plant species, their pollinators and their seed dispersers. In these networks, pollinators and seed dispersers form an indirect plant-mediated mutualism [10] because both benefit each other by increasing the reproductive output and dispersal capacity of the shared food plant. We study these coupled mutualistic networks in Europe’s last relict of old-growth lowland forest (Białowieża, Poland) [11] , and find strong evidence that plants mediate a correlated response of both their pollinators and their seed dispersers to the degradation of this forest ecosystem. Thus, habitat degradation may critically endanger the integrity of ecosystems through a parallel loss of multiple animal-mediated ecosystem services. Overall effects of logging and fragmentation We quantified the interactions between the focal plants and their animal mutualists in the last European relict of old-growth lowland forest in Białowieża, eastern Poland [11] . During the last century, this unique ecosystem has been fragmented, and over 80% of the Polish part of the forest (625 km 2 ) has been converted to secondary forests owing to commercial logging [12] . Currently, only 45 km 2 of the forest still feature natural dynamics typical of old-growth forests. In this setting, we established 17 study sites scattered over 400 km 2 , situated in both logged and old-growth forests and covering various landscape contexts ranging from forest interior to edges to small forest remnants. In a 2-year field survey on these sites, we quantified the mutualistic interactions of the focal plant species with both their pollinators and their seed dispersers. We documented 5,784 interactions with 294 pollinator species (mainly from the orders Diptera, Hymenoptera, Coleoptera and Lepidoptera) and 5,935 interactions with 34 seed disperser species (30 avian and 4 mammalian species; Fig. 1 ). Rarefaction analyses indicated that our sampling identified the functionally most important species ( Supplementary Fig. 1 ). Based on this data set, we quantified the number of partners (number of distinct links) and the interaction frequency (rate of interactions) of the plants for both mutualistic relationships. Both the number of partners and interaction frequency are major determinants of a species’ impact in an interaction network [13] , [14] . The number of partners is essential for species persistence [13] , and the interaction frequency is highly correlated with the effect of interacting species on each other’s reproductive performance [14] , [15] , [16] . 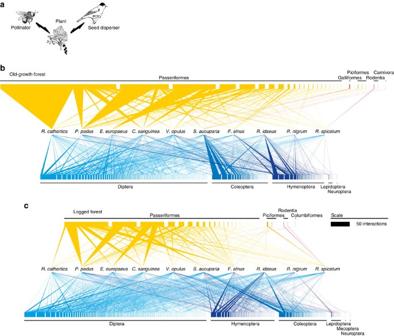Figure 1: Coupled mutualist networks of plants and their pollinators and seed dispersers in old-growth forest and logged forest in Białowieża (Poland). (a) A simple association of a plant, a pollinator and a seed disperser. (b,c) The quantified networks in old-growth forest (b) and logged forest (c). The 10 focal plant species are in the centre of each depicted network, pollinators are at the bottom and seed dispersers are at the top. Each bar depicts an animal species and its width represents its mean abundance across the two study years. The widths of the base of the lines connecting plants with their pollinators and seed dispersers depict pair-wise interaction frequencies. SeeSupplementary Table 6for full species names. Figure 1: Coupled mutualist networks of plants and their pollinators and seed dispersers in old-growth forest and logged forest in Białowieża (Poland). ( a ) A simple association of a plant, a pollinator and a seed disperser. ( b , c ) The quantified networks in old-growth forest ( b ) and logged forest ( c ). The 10 focal plant species are in the centre of each depicted network, pollinators are at the bottom and seed dispersers are at the top. Each bar depicts an animal species and its width represents its mean abundance across the two study years. The widths of the base of the lines connecting plants with their pollinators and seed dispersers depict pair-wise interaction frequencies. See Supplementary Table 6 for full species names. Full size image Model selection suggested that changes in both the number of partners and interactions of plants in both mutualisms were consistently associated with logging of old-growth forests ( Fig. 1 ; Table 1 ; and Supplementary Table 1 ). Forest fragmentation was of minor importance ( Table 1 ), which may be explained by the moderate degree of fragmentation and the diverse mosaic of forest and open landscape in our study area. This adds to previous findings that predict moderate habitat fragmentation to be of lesser importance than typically observed levels of habitat degradation [17] , [18] . Table 1 Summary of model selection. Full size table We used the predictions derived from the most parsimonious models ( Table 1 ) and calculated for each plant species i the proportional difference in the number of partners and interactions for each mutualism j between the mean of old-growth forest and logged forest as the log-response ratio, LR ij =ln( y ij (Logged) / y ij (Old-growth) ) (see Methods section) [19] . This unitless metric allows us to test for a significant change in the number of partners and interactions with logging when averaged across all plant species. Logging, averaged across all plant species, had contrasting effects on the number of partners and interactions of plants in the two mutualisms ( Fig. 2a,b ; and Table 1 ). Logging caused an average increase of 18% in the number of partners in plant–pollinator associations ( t -test, t =7.03, n =10, P <0.001; Fig. 2c ), and a decrease of 27% in the number of partners in plant–seed disperser associations ( t -test, t =−4.64, n =10, P <0.01; Fig. 2c ). Logging had no consistent effect on interaction frequencies of plants with pollinators (average change of 4.7%; t -test, t =0.961, n =10, P >0.05; Fig. 2d ), but reduced interaction frequencies with seed dispersers by 50% ( t -test, t =−4.11, n =10, P <0.01; Fig. 2d ). The increased number of pollinator species in logged forest may derive from local disturbance regimes associated with logging that increase the availability of open habitats and alternative resources [20] . Conversely, the substantial loss of partners and interactions in the plant–seed disperser associations can at least partly be attributed to a loss of forest specialists that rely on old-growth forests [21] . A previous study has shown that the loss of forest specialists in logged forests reduces the redundancy in these plant–seed disperser associations [21] . These changes in interaction structure are likely to limit the dispersal and recruitment ability of fleshy-fruited plants in secondary forest habitats [15] , [22] . Thus, our study supports previous concerns on the high vulnerability of animal-mediated seed dispersal to habitat degradation [18] , [23] . 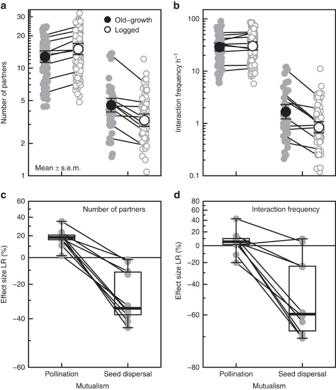Figure 2: Effects of logging on the number of partners and interactions of plants in the plant–pollinator and plant–seed disperser mutualisms. The number of partners (a) and the interaction frequency (b) of plants in both mutualisms (plant–pollinator and plant–seed disperser) in old-growth forest (closed circles) and logged forest (open circles). Grey circles depict model predicted data (n=322), lines represent the predicted mean response of each of the 10 focal plant species, and black circles indicate the predicted mean response on the level of the plant assemblage (mean±s.e.m.). The LR ratios (LRs) inc,destimate the ‘effect size’ of logging. LR measures the proportional difference between the mean value of the response variableyin old-growth forest and the mean value ofyin logged forest. LR<0 indicates a negative effect of logging on (c) the number of partners and (d) interaction frequency of plants in both mutualisms. The lines inc,dconnect the responses of both mutualisms for each plant species. Figure 2: Effects of logging on the number of partners and interactions of plants in the plant–pollinator and plant–seed disperser mutualisms. The number of partners ( a ) and the interaction frequency ( b ) of plants in both mutualisms (plant–pollinator and plant–seed disperser) in old-growth forest (closed circles) and logged forest (open circles). Grey circles depict model predicted data ( n =322), lines represent the predicted mean response of each of the 10 focal plant species, and black circles indicate the predicted mean response on the level of the plant assemblage (mean±s.e.m.). The LR ratios (LRs) in c , d estimate the ‘effect size’ of logging. LR measures the proportional difference between the mean value of the response variable y in old-growth forest and the mean value of y in logged forest. LR<0 indicates a negative effect of logging on ( c ) the number of partners and ( d ) interaction frequency of plants in both mutualisms. The lines in c , d connect the responses of both mutualisms for each plant species. Full size image Correlated loss of interactions In the next step, we used the LR ratios (LR ij ) to test whether effects of logging on interactions of plant species with their pollinators and their seed dispersers were correlated. From previous work we know that phylogenetically related species tend to interact with a similar set of mutualistic partners, because ecological interactions are evolutionarily conserved [24] , [25] . Thus, we can expect that, owing to shared mutualistic partners, interactions of closely related plant species should be affected more similarly by perturbation than interactions of distantly related species [24] . To account for this effect of phylogenetic relatedness, we used correlations based on phylogenetic independent contrasts (PICs; see Methods section) [26] . After accounting for phylogenetic relationships among plant species, we found a strong and significant correlation between the responses of both mutualisms to logging (Pearson’s correlation forced through origin, number of partners: r =0.72, one-tailed P <0.01; interaction frequency: r =0.73, one-tailed P <0.01, n =9 in both cases; Fig. 3b,c ). The correlated response of both mutualisms to logging was also supported by non-phylogenetic correlations by raw data and by randomization tests ( Supplementary Table 2 ; and Supplementary Figs 2 and 3 ). This suggests that independently of the similarities in interactions because of the shared ancestry of plants, stronger changes in one mutualism were correlated with changes in the other mutualism because both are ‘biologically coupled’ through the reproductive cycle of the plants. Perhaps the most striking aspect of these results is that we found this correlation despite the apparently contrasting effects of logging on pollinators and seed dispersers. Previous studies that used single plant species as model organisms also have found contrasting effects of habitat degradation on pollinators and seed dispersers [27] . These studies concluded that different functional groups of animals respond idiosyncratically to land-use change. However, our study revealed hidden effects of land-use changes on the structure of ecological communities. Such effects will most likely remain undetected in studies that do not simultaneously quantify different types of species interactions on the level of entire communities. 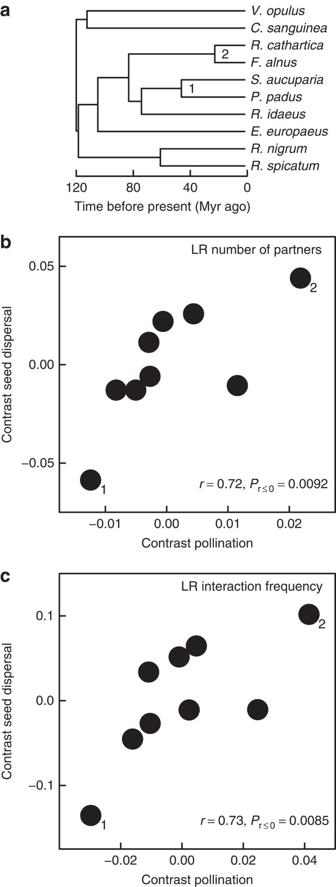Figure 3: Correlations between the responses of pollinators and seed dispersers to logging. Phylogenetic relationships of the focal plant species (a) with branch lengths given in million years (Myr). Correlations between phylogenetic independent contrasts (PICs;n=9) of the LR ratios (LRs) of (b) the number of partners and (c) the interaction frequency of plants in the plant–pollinator and plant–seed disperser mutualisms. Highlighted are the contrasts (nodes 1 and 2 in the phylogeny) of two closely related species pairs (1:Prunus padusandSorbus aucuparia; 2:Frangula alnusandRhamnus cathartica). Figure 3: Correlations between the responses of pollinators and seed dispersers to logging. Phylogenetic relationships of the focal plant species ( a ) with branch lengths given in million years (Myr). Correlations between phylogenetic independent contrasts (PICs; n =9) of the LR ratios (LRs) of ( b ) the number of partners and ( c ) the interaction frequency of plants in the plant–pollinator and plant–seed disperser mutualisms. Highlighted are the contrasts (nodes 1 and 2 in the phylogeny) of two closely related species pairs (1: Prunus padus and Sorbus aucuparia ; 2: Frangula alnus and Rhamnus cathartica ). Full size image Bottom-up control Previous studies highlight the importance of shifts in the density of plant resources in degraded habitats as determinants of the direction and magnitude of land-use effects on mutualistic plant–animal interactions [15] , [20] , [28] , [29] . Although pollinators and seed dispersers differ in their specialization on food plants [30] , both may respond similarly to changes in the densities of the plants [9] , [10] , [31] . Accordingly, path analyses revealed that shifts in plant population densities between old-growth forest and logged forest largely explained the magnitude of the effects of logging on interactions of plants with their pollinators and seed dispersers ( Fig. 4 ): plant species that showed a disproportionate increase or decrease in their density in logged forest also experienced a disproportionate gain or loss of partners and interactions in both mutualistic relationships. These results suggest that effects of habitat degradation on mutualistic plant–animal interactions are bottom-up-controlled by shifts in the density of food plants that occur following habitat degradation [10] . This does not necessarily mean that shifts in species interactions follow the exact trajectories of shifts in the population density of plants, as is evident from our results ( Fig. 2c,d ). Our results rather suggest that shifts in the population density of plant resources are likely to amplify the magnitude of the effects of habitat degradation on species interactions. 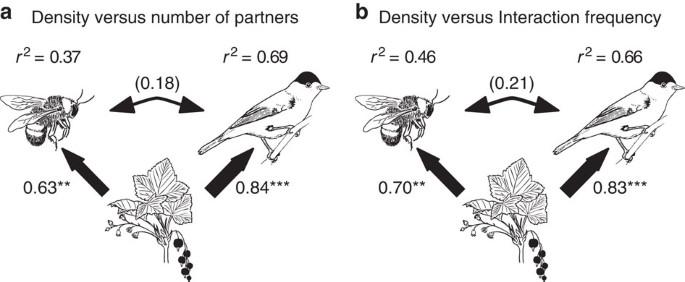Figure 4: Summary of path analyses testing for bottom-up control in the responses of pollinators and seed dispersers to logging. Path models are based on phylogenetic independent contrasts (PICs;n=9) and show the effects of the LR ratio (LRij) in plant density between old-growth forest and logged forest on the LR ratio in number of partners (a) and interaction frequencies (b) of plants in the plant–pollinator and plant–seed disperser mutualism. Shown are results for the predicted data from most parsimonious linear mixed-effects models (Table 1). Standardized path coefficients are given next to path arrows. Arrow widths are proportional to path coefficients. Residual covariance is denoted by double-headed arrows. Proportion of explained variance (r2) is denoted above each mutualism. Significance of path coefficients is depicted by **P<0.01 and ***P<0.001. Both path models fit the data (a)χ2=1.5, df=2,P=0.47; (b)χ2=2.19, df=2,P=0.33. Figure 4: Summary of path analyses testing for bottom-up control in the responses of pollinators and seed dispersers to logging. Path models are based on phylogenetic independent contrasts (PICs; n =9) and show the effects of the LR ratio (LR ij ) in plant density between old-growth forest and logged forest on the LR ratio in number of partners ( a ) and interaction frequencies ( b ) of plants in the plant–pollinator and plant–seed disperser mutualism. Shown are results for the predicted data from most parsimonious linear mixed-effects models ( Table 1 ). Standardized path coefficients are given next to path arrows. Arrow widths are proportional to path coefficients. Residual covariance is denoted by double-headed arrows. Proportion of explained variance ( r 2 ) is denoted above each mutualism. Significance of path coefficients is depicted by ** P <0.01 and *** P <0.001. Both path models fit the data ( a ) χ 2 =1.5, df=2, P =0.47; ( b ) χ 2 =2.19, df=2, P =0.33. Full size image Our study provides one of very few empirical examples of coupled, interdependent networks [7] , [32] , [33] , [34] , [35] , [36] . Together with the existing examples, our study highlights that complex systems, be it infrastructural [33] , biological [34] or climate systems [35] , do not exist in isolation but form parallel, interdependent networks that respond collectively to perturbation. Our study demonstrates that strong interdependence among coupled networks can cause predictable transmission of perturbations across these networks. This suggests that it may be essential to consider this interdependence, if we aim to identify properties that account for the structural and functional stability of complex networks. The ecological implications of our study are twofold. First, our results demonstrate that a consideration of the biotic context [29] of mutualistic associations (for example, shifts in resource densities) improves predictions of the effects of land-use changes on species interactions. Second, we find that habitat degradation induces a correlated shift in the interaction structure of the studied plant species and their animal mutualists. These results suggest that effects of habitat degradation on multiple interdependent plant–animal mutualistic networks are predictable. In principle, our findings may also be valid for other trophic interactions directly or indirectly linked to plant resources (for example, plant–herbivore or plant–herbivore–parasitoid webs) [7] , [10] . As old-growth forests comprise only 0.2% of all extant European forests [37] and are globally declining, our findings signal an alarm, as they predict that the conversion of primary old-growth forest ecosystems to secondary habitats may involve a parallel loss of multiple animal-mediated ecosystem services. Study area We conducted our field campaign in the Białowieża Forest, the best-preserved European old-growth lowland forest, extending across the border between Poland and Belarus [38] , [39] . On Polish territory, the forest covers an area of ~625 km 2 . Within the Białowieża National Park (~105 km 2 ), an area of ~60 km 2 is strictly protected and an area of ~45 km 2 features natural vegetation dynamics typical for old-growth forests without recent human influence [40] , [41] . Over 80% of the remaining forest has been shaped by commercial logging since the First World War [38] , [39] . Moreover, most riverine areas of the forest had been cleared during the 16th and 17th centuries for hay production, which resulted in a mosaic of meadows along rivers and in the vicinity of villages [41] . The core of the Białowieża National Park is an exceptional and unique reference site for studying the impact of anthropogenic habitat degradation on ecological processes in temperate forest ecosystems [38] , [39] , [40] , [41] . Study species and design We focussed our study on woody, fleshy-fruited plant species that depend on animal pollination and seed dispersal (see below). As the focal plant species of our study are mainly associated with ash–alder floodplain forests ( Fraxino – Alnetum community) [42] , we chose our study sites within this plant association. In 2011, we established 10 study sites in the interior ( n =3) and at edges ( n =2) of logged forest (stand age: ~50 years) and in the interior ( n =2) and at edges ( n =3) of old-growth forest within the national park (stand age: ~100–150 years). In 2012, we established additional study sites at edges ( n =3) and in fragments ( n =4; size ~1 ha) of logged forest to extend the fragmentation gradient. Study sites in the forest interior were located at least 500 m from forest edges, and forest edge sites were located at transitional zones between closed forest and riverine meadows. Forest fragment sites were located in small ash–alder forest remnants entirely surrounded by meadows (for details on characteristics of the study sites, see Supplementary Tables 3 and 4 ). Thus, our study was conducted on a total of 17 sites scattered over ~400 km 2 covering two-thirds of the Polish part of the Białowieża Forest. The pair-wise distance between study sites ranged from 1.4 to 23 km (11±5.8 km, mean±s.d.). We searched for fleshy-fruited plant species in a radius of 500 m around the centre of each study site and identified 16 plant species. For the analyses, we selected the subset of plant species that occurred in both logged and old-growth forest habitats, as well as in both continuous (interior) and fragmented (edge and fragment) forest habitats. Thus, the data set included 10 understorey, woody, fleshy-fruited plant species from nine genera and five families (five tree and five shrub species, respectively; Supplementary Table 5 ). These plant species are common throughout Europe [43] . In ash–alder floodplain forests, these plant species occur in high densities and thus represent critical keystone species for flower-visiting insects and frugivorous birds and mammals. Sampling of pollinator assemblages From May to June in 2011 and 2012, we monitored the flowering of the focal plant species on the study sites weekly ( Supplementary Table 5 ). According to the availability of flowering individuals, we selected three ( n =78), two ( n =74) or one individual ( n =35) per species for the pollinator observations per study site and year. To document pollinator visits on flowers, we observed each species on each study site twice for 30 min in 2011 and three times for 15 min in 2012 (2011: 60 min per plant species per study site; 2012: 45 min × per plant species × per study site). Flower-visiting insects were sampled between 9:00 and 17:30 hours during good weather conditions and simultaneously at different study sites (three observers in 2011 and two observers in 2012). Because of potential temporal differences in pollinator activity, we varied the time of day in which sampling took place across sites and across the sessions for each species per site. We conducted one session in the morning (9:30–12:30 hours), one in the early afternoon (12:30–15:30 hours) and one in the late afternoon (15:30–17:30 hours). During each sampling session, all insect visitors that contacted floral sexual organs were caught with a sweep net and killed in ethyl acetate in a test tube. In the case of larger plant individuals (that is, trees or large shrubs), we restricted our sampling to a subset of flowers. Hence, for large plant individuals, the sampling sessions represent a random snapshot of simultaneous flower visitor activity on plants. In the subsequent analyses, we accounted for the uncertainties associated with our sampling protocol (see below). In the first study year, we sorted all caught insects, identified them to the lowest taxonomic level possible, and prepared a collection of reference specimens (with the help of two experts; see Acknowledgements section). In the second year, we extended this reference collection and used it for identification of caught insects. We identified 76% of all flower visitors to the species level, 88% to the genus level and 95% to the family level (for simplicity, we refer to all morphospecies as species). All flower visitors were assumed to be potential pollinators (hereafter referred to as pollinators). In total, we accumulated 157 h of pollinator observations (66 h in 2011 and 91 h in 2012), distributed over 81 days (34 days in 2011 and 47 days in 2012). After each sampling session, we counted the number of observed flowers as well as the total flower burden of each observed plant individual. In the case of trees, we counted the flowers on representative parts of the tree and extrapolated over the whole crown. For analyses, we calculated the mean flower burden across the observed individuals of each plant species on each study site per year. Total flower burden and number of observed flowers were highly correlated (Pearson’s r =0.81, n =187, P <0.001). The results of subsequent analyses (see below) were similar for both measures; thus, we only report results of the analyses based on the number of observed flowers. Sampling of seed disperser assemblages From July to October in 2011 and 2012, we monitored fruit ripening of the plant species on the study sites weekly ( Supplementary Table 5 ). According to the availability of fruiting individuals, we selected three ( n =91), two ( n =24) or one individual ( n =21) per species for the frugivore observations on each study site per year. We observed each species on each study site and year three times for 6 h starting at sunrise (18 h × per plant species × per study site × per year). We observed plant–frugivore interactions with binoculars from camouflaged tents simultaneously at different study sites (7 observers in 2011 and 14 observers in 2012). We recorded all frugivore species visiting the individual plants, as well as the number of frugivore individuals, duration of visits and their fruit-handling behaviour (for details, see ref. 21 ). In total, we accumulated 2,430 h of seed disperser observations (702 h in 2011 and 1,728 h in 2012), distributed over 158 days (67 days in 2011 and 91 days in 2012). After each sampling session, we counted the fruits of the observed plant individuals. For trees, we counted the fruits on representative parts of the tree crown and then extrapolated over the whole tree crown. For analyses, we calculated the mean number of fruits across the observed individuals for each plant species on each study site per year. Sampling of plant population densities We recorded the abundance of fleshy-fruited plant species on 13 of the 17 study sites ( Supplementary Table 3 ). To do so, we established 20 alternating squares on 10 of the study sites and, owing to logistical constraints, 10 squares on 3 of the sites, each 20 × 20 m (covering a total area of 0.8 or 0.4 ha, respectively, on each study site). In each square, we counted the number of individuals of each focal plant species. Because all of the focal plant species were perennials, we assumed that their population abundance would not change significantly between years. Thus, although we studied interactions with pollinators and seed dispersers in two consecutive seasons (2011 and 2012), we estimated plant abundances only in the second season (2012). We used the mean density per species per square as an estimate of absolute population density. Statistical analysis We used linear mixed-effects models to analyse the variation in the number of partners and interaction frequency of plants in the plant–pollinator and plant–seed disperser mutualisms. In these analyses, we treated fragmentation (interior, edge and fragment), logging (logged and old-growth) and mutualism (plant–pollinator and plant–seed disperser) as fixed factors. We refined comparisons of fragmentation using orthogonal contrasts to compare between continuous and fragmented forest (interior versus edge and fragment) and among fragmented forests (edge versus fragment). As our design is not full factorial with respect to logging and fragmentation, we only included interactions of logging × mutualism and fragmentation × mutualism but not the logging × fragmentation interaction. Furthermore, our study design was not full factorial with respect to site, year and plant species (that is, not all plant species occurred on every study site and not all study sites were sampled in both years). Therefore, we fitted site, year and plant species as separate random grouping factors. We nested mutualism within plant species, corresponding to a full factorial design. To account for any potential effects of differences in sampling intensity of pollinator assemblages in 2011 and 2012 (60 min versus 45 min), we used the relative sampling duration (sampling intensity) as an offset [44] , [45] in the models (coded for pollinators: 1 in 2011 and 0.75 in 2012; seed dispersers: 1 in both years). Furthermore, we included the abundance of resource units (flowers or fruits) as a continuous covariate in the models to account for variation in resource abundance across focal plants. Number of partners, interaction frequency and number of resource units were transformed to their natural logarithm before statistical analyses. Based on the above-described global models, we generated a set of component models. This model set contained 25 component models for all possible combinations of predictor variables plus a model including only the intercept (the offset was kept fixed). To find the most parsimonious model, these models were compared according to small sample unbiased Akaike’s information criterion (AIC c ; Supplementary Table 1 ). To obtain a measure of the relative importance of the main predictors, we calculated the Akaike weight for each model and summed these weights for each predictor over all models including the respective variable [46] . Significance of the fixed effects in the most parsimonious models was assessed using a bootstrap procedure with 10,000 simulations as implemented in the R package lme4 refs 47 , 48 . The decision to use log-transformed response variables may influence the results of our analyses [45] . Thus, we compared both models to alternative generalized models assuming a Poisson distribution for the number of partners (discrete counts of species), and a Gamma distribution for the interaction frequency (continuous rate of interaction per hour; Supplementary Methods ). The results of the generalized models confirmed those of the models based on the log-transformed response variables. However, as the models based on the log-transformed response variables had substantially higher prediction accuracy and a slightly higher precision than the generalized models ( Supplementary Fig. 5 ), we report results of the models based on the log-transformed data. The most parsimonious models suggested that logging, but not fragmentation, explained changes in the interaction structure of plants with their pollinators and seed dispersers ( Table 1 and Supplementary Table 1 ). Thus, we used these models to predict the number of partners and interactions of the plants in both mutualistic relationships in logged and old-growth forest (at the level of observations). We conditioned these predictions on the specified random effects [47] . Furthermore, to account for any potential effects of differences in sampling intensity of pollinator assemblages between study years, we explicitly incorporated these differences into the predictions (that is, by setting the sampling effort in both years to the same relative intensity of 1). For comparison, we ran all subsequent analyses based on the predicted data and based on the raw data. The estimated effects based on the raw data were equal or stronger compared with those based on the predicted data ( Supplementary Fig. 2 ; and Supplementary Table 2 ), suggesting that the estimates based on the predicted data are conservative. In the main text, we report the results based on the more conservative model predictions that explicitly integrate potential effects of sampling intensity. Based on these predictions, we calculated for each plant species i the mean number of partners and interactions in old-growth forest and logged forest in the pollination and seed dispersal mutualisms. In the next step, we used the mean values of the number of partners and interactions of plant species i in mutualism j to calculate the LR ratio between old-growth forest and logged forest as LR ij =ln( y ij (Logged) / y ij (Old-growth) ) [19] . LR ratios are the most adequate metric for our purpose because they estimate a proportional difference between habitats that can be readily compared between plant species, and because they have sampling properties that are known to be normal and that are robust to bias from small sample sizes [19] . To facilitate the interpretation of the results, we transformed the axes of the LR ratios in Fig. 2 to an index of percentage change (%)=–(1− e LR ) × 100 (ref. 19 ). However, statistical analyses were performed using untransformed LR ratios. We used the LR ratios for a prediction of the expected change in number of partners and interaction frequencies across the studied plant species due to logging, and used t -tests to evaluate the null hypothesis of no change between old-growth forest and logged forest. Furthermore, we used more conservative binomial tests to test whether the raw effect directions were consistent across the ten plant species. The results of the binomial tests were consistent with those of the t -tests. Test for correlated response of both mutualisms We used correlations to test whether the responses of both mutualisms to logging (LR ij ) were correlated across the focal plant species. As pollinators and seed dispersers form an indirect plant-mediated mutualism [10] , we can expect a positive correlation between the effects of logging on interactions in both mutualisms [31] and used one-tailed statistical tests in all subsequent analyses. As the 10 studied plant species are part of a hierarchically structured phylogeny, we calculated correlations using PICs [26] , [49] . We extracted the appropriate information from a dated phylogeny of a large European flora ( Fig. 3a ) [50] . Phylogenetic correlations were computed through the origin [51] . We used generalized least squares to estimate the strength of the phylogenetic signal (Pagel’s λ ) [26] , [52] . As the likelihood profiles of the estimates were flat, we used the special cases with λ set to zero (a star phylogeny) and with λ set to 1 (Brownian motion) [52] . As the sample size for two plant species ( Rubus idaeus and Cornus sanguinea ; Supplementary Table 5 ) was limited, we performed generalized least squares analyses with and without weighting of the LR ratios of plant species by their variance, giving greater weight to plant species with higher ‘certainty’. Weighted and unweighted analyses led to identical conclusions ( Supplementary Table 2 ). Finally, we used a permutation test to assess whether the observed correlations were larger than expected from a null distribution (assuming no relationship between the responses of both mutualisms). In this test, we randomized the LR ratios in one mutualism among the tips of the phylogeny (999 permutations), recalculated PICs and correlation coefficients, and compared the resulting null distribution with the observed correlation coefficients. Observed correlations were significantly larger than expected from the null distribution ( Supplementary Fig. 3 ). Test for bottom-up control We used path analyses to test whether effects of logging on both mutualisms were bottom-up-controlled by specific shifts in plant densities between old-growth forest and logged forest. First, we calculated the LR ratio of plant population densities between old-growth forest and logged forest, and calculated PICs (similar to the responses of both mutualisms). As we only had vegetation data from 13 of the 17 study sites, we repeated the above-described analytical procedures only including these 13 sites and recalculated LR ratios for both mutualisms. The results based on the full and reduced data sets were qualitatively and quantitatively similar. Then we constructed a priori path models to test for bottom-up control based on the PICs ( Fig. 4 ). These models included the correlations of the PICs of the LR plant density on the PICs of the LR in number of partners and LR in interaction frequencies in both mutualisms (plant–pollinator or plant–seed disperser). We also included the covariance between both mutualisms. We calculated correlations in the path models through the origin [51] . Model fit was assessed with a χ 2 -test. Path analyses based on model predicted data and raw data led to the same conclusion that the correlated effects of logging on both mutualisms were mediated by shifts in the density of plant populations on logged sites ( Fig. 4 ; and Supplementary Fig. 4 ). Spatial autocorrelation We are aware that our study design is limited to a single relict of preserved primary old-growth forest within the Białowieża National Park, which is surrounded by logged forest. Therefore, we tested for spatial dependency (Moran’s I similarity) in the residuals of the two most parsimonious models. For both models, Moran’s I similarities were close to zero and did not decrease with increasing distance (0–24 km) of discrete distance classes (2 km), which indicated a random spatial pattern ( Supplementary Fig. 6 ). Statistical software All analyses were conducted in R [53] using the packages lme4 (ref. 47 ) and glmmADMB [54] for analysing mixed-effects models, MuMIn [55] for model selection, packages ape [56] and nlme [57] for phylogenetic analyses and package lavaan [58] for path analyses. Networks were plotted with a customized version of the function plotweb from the package bipartite [59] . How to cite this article: Albrecht, J. et al. Correlated loss of ecosystem services in coupled mutualistic networks. Nat. Commun. 5:3810 doi: 10.1038/ncomms4810 (2014).